Mettl3-mediated m6A RNA methylation regulates the fate of bone marrow mesenchymal stem cells and osteoporosis N 6 -methyladenosine (m 6 A) is the most abundant epigenetic modification in eukaryotic mRNAs and is essential for multiple RNA processing events during mammalian development and disease control. Here we show that conditional knockout of the m 6 A methyltransferase Mettl3 in bone marrow mesenchymal stem cells (MSCs) induces pathological features of osteoporosis in mice. Mettl3 loss-of-function results in impaired bone formation, incompetent osteogenic differentiation potential and increased marrow adiposity. Moreover, Mettl3 overexpression in MSCs protects the mice from estrogen deficiency-induced osteoporosis. Mechanistically, we identify PTH (parathyroid hormone)/Pth1r (parathyroid hormone receptor-1) signaling axis as an important downstream pathway for m 6 A regulation in MSCs. Knockout of Mettl3 reduces the translation efficiency of MSCs lineage allocator Pth1r, and disrupts the PTH-induced osteogenic and adipogenic responses in vivo. Our results demonstrate the pathological outcomes of m 6 A mis-regulation in MSCs and unveil novel epitranscriptomic mechanism in skeletal health and diseases. Bone marrow mesenchymal stem cells (MSCs) are the common progenitors for osteoblasts and marrow adipocytes. The reciprocal balance between osteogenic and adipogenic differentiation of MSCs is under tightly spatiotemporal controls to safeguard skeletal health [1] , [2] , [3] . Aged-related osteoporosis is featured with low bone mass and excessive accumulation of adipose tissue in bone marrow milieu [1] , [2] , [3] . Under aging or other pathological stimuli such as hormone disorders, the bone marrow MSCs undergo preferential shift of differentiation towards adipocytes, resulting in the increase in marrow adiposity and progressive bone loss [1] , [4] , [5] . These alterations in bone micro-architecture lead to the increased skeletal fragility and susceptibility to fracture. However, the explicit mechanisms under which the lineage allocation of MSCs favors adipogenic to osteogenic lineage remain unclear. N 6 -methyladenosine (m 6 A) is the most prevalent post-transcriptional internal mRNA modification that regulates the fine-tuning of a variety of biological processes [6] , [7] , [8] . In mammals, m 6 A is catalyzed by the methyltransferase complex consisting of an enzymatic subunit METTL3, a substrate recognition subunit METTL14 and a regulatory subunit WTAP [9] , [10] , [11] , and it can be erased by demethylases FTO and ALKBH5 [12] , [13] . At molecular level, m 6 A marks are dynamically installed and removed from their regulated transcripts to adjust RNA metabolisms, including alternative splicing, RNA stability, and translation, in response to multiple signaling cues during normal cellular processes or under stress or diseases [14] , [15] , [16] , [17] , [18] , [19] . Alterations in expressions of m 6 A methylated transcripts subsequently affect the cellular function, identity and stemness of their residing cells [20] , [21] , [22] , [23] , [24] , determining cell fate in a context-dependent manner. Recent in vivo studies made great breakthroughs in deciphering the intriguing involvement of m 6 A in mammalian development. Aberrant m 6 A levels upon Mettl3 and/or Mettl14 deficiency attenuated cell cycle progression, and disrupted the proper lineage commitment and differentiation of functional stem cells, resulting in retarded neurogenesis, immune defects, and infertility [25] , [26] , [27] , [28] . Given the strong correlation of m 6 A with health and diseases, we focus on exploring the potential involvement of m 6 A in bone homeostasis, about which little was known. By generating conditional knockout and knock-in mutant mice, we unveil a crucial effect of m 6 A functioning in modulating MSCs differentiation, and discover PTH/Pth1r signaling axis as an important m 6 A downstream mechanism pathway. Our findings provide a new insight in the pivotal regulatory role of m 6 A in skeletal health and diseases. Conditional deletion of Mettl3 in MSCs leads to low bone mass and high marrow adiposity To study the potential role of Mettl3 in bone marrow MSCs lineage allocation and bone diseases, we first examined the expression of Mettl3 in mouse bone tissues. Immunostaining showed that Mettl3 is prevalently expressed in the bone cells and bone marrow of mice, but absent in chondrocytes of the growth plate zone (Supplementary Fig. 1 ). Since genomic Mettl3 knockout is embryonic lethal [20] , we generated Mettl3 flox ( Mettl3 fl /+ ) mice using CRISPR/Cas9 technique (Supplementary Fig. 2a ), and then bred Mettl3 fl /+ mice with Prx1-Cre transgenic mice to obtain conditional homozygous Mettl3 knockout mice, Prx1-Cre;Mettl3 fl/fl mice, as well as heterozygous Mettl3 knockout mice, Prx1-Cre;Mettl3 fl/+ mice (Supplementary Fig. 2b,c ). Prx1-Cre;Mettl3 fl/fl mice were viable, though with a lower survival rate (Supplementary Fig. 2d ), and exhibited a sex bias towards maleness (about 4.5:1), in consistent with previous studies [17] , [29] . They had smaller size, lighter weight and retarded growth features compared to their Mettl3 fl/fl control littermates at 4 weeks of age. Immunostaining of femur paraffin sections and western blot analysis proved the deletion of Mettl3 was successful, which subsequently reduced the m 6 A level in MSCs (Supplementary Fig. 2e-g ). Micro-computed tomography (μCT) analysis of trabecular bone of the distal femur metaphysis revealed that bone mineral density (BMD) and bone volume/tissue volume ratio (BV/TV) were significantly reduced in Prx1-Cre;Mettl3 fl/fl and Prx1-Cre;Mettl3 fl/+ male mice compared to their Mettl3 fl/fl littermates (Fig. 1a, b ). In addition, Mettl3 deletion also diminished the trabecular number (Tb.N), trabecular thickness (Tb.Th) and midshaft cortical thickness (Ct.Th), while increasing the trabecular separation (Tb.Sp) (Fig. 1b ). Von Kossa staining of the undecalcified sections further confirmed the low bone mass phenotype of Prx1-Cre;Mettl3 fl/fl mice (Fig. 1c ). Moreover, the Mettl3 conditional knockout mice had slower mineral apposition rate (MAR) and bone formation rate (BFR), with also less osteoblast number (N.Ob/B.Pm) (Fig. 1e ), suggesting that deletion of Mettl3 in MSCs contributed to the impaired bone formation in mice. We also observed a more active osteoclast state in Prx1-Cre;Mettl3 fl/fl mice (Fig. 1d, e ), supporting a faster bone tissue breakdown occurring in the Mettl3 conditional knockout mice. Mettl3 knockout only led to a slightly yet not significantly shortened growth plate and hypertrophic zones (Supplementary Fig. 3 ). Fig. 1 Deletion of Mettl3 in MSCs leads to low bone mass and high marrow adiposity. a Representative μCT images of distal femurs and midshaft cortical bone. Scale bar, 500 μm. b Quantitative μCT analyses of distal end of femurs ( n = 8). c Von Kossa staining of undecalcified sections of femurs. Scale bar, 500 μm. d TRAP staining of femur sections. Scale bar, 50 μm. e Histomorphometric analyses of trabecular bone from the femur metaphysic ( n = 8). f Immunohistochemical staining of FABP4. Scale bar, 50 μm. g Number and area of adipocytes in the distal marrow per tissue area ( n = 8). Data are expressed as mean ± s.e.m. ; * P < 0.05, ** P < 0.01, *** P < 0.001 by one-way ANOVA with Tukey’s post hoc test Full size image Interestingly, we observed that the loss of bone mass is associated with apparently increased bone marrow adipose tissue (MAT) accumulation in the Prx1-Cre;Mettl3 fl/fl mice (Fig. 1f ). Both the number and the density of marrow adipocytes were elevated in Prx1-Cre;Mettl3 fl/fl mice compared to their Mettl3 fl/fl controls (Fig. 1g ). Overall, the skeletal manifestations of Mettl3 conditional knockout mice resemble the pathological phenotypes of osteoporosis, implying a lineage allocation disorder in MSCs with low m 6 A methylation level. Loss of Mettl3 in MSCs leads to compromised osteogenic potential and increased adipogenic differentiation Next, we isolated MSCs from Mettl3 fl/fl and Prx1-Cre;Mettl3 fl/fl mice to verify their osteogenic and adipogenic potentials in vitro. The incompetent osteogenic differentiation ability of Mettl3 deleted MSCs was evidenced by weaker alkaline phosphatase staining (ALP) activity and less calcium mineralization (Fig. 2a ), and the downregulated expression of osteogenic markers, including Runx2 , Sp7 , Alp , and Bglap (Fig. 2b ). On the contrary, the increased intensity of oil red O staining (Fig. 2c ) and significantly elevated expression of adipogenic factors, including Pparγ , Cebpα , Adipoq , Plin1 , and CD36 (Fig. 2d ), demonstrated the enhanced adipogenic potential of Prx1-Cre;Mettl3 fl/fl MSCs. Fig. 2 Mettl3 -deficient MSCs exhibit compromised osteogenic potential and increased adipogenic differentiation. a Representative images and quantitative analyses of ALP and ARS staining of MSCs isolated from Mettl3 fl/fl and Prx1-Cre;Mettl3 fl/fl mice. b qRT-PCR analyses of the expression of Runx2 , Sp7 , Alp and Bglap under osteogenic condition. c Representative images and quantitative analysis of oil red O staining. Scale bar, 100 μm. d qRT-PCR analyses of the expression of Cebpα , Pparγ , Adipoq, Plin1 , and CD36 under adipogenic condition. Results are from three independent experiments. Data are expressed as mean ± s.e.m. ; * P < 0.05, ** P < 0.01, *** P < 0.001 by two-tailed Student’s t test Full size image Deletion of Mettl3 in Lepr + MSCs results in bone impairment and marrow fat accumulation We next sought to examine whether Mettl3 has comparable importance in a later stage of bone formation. To this end, we used Lepr-Cre line, which mainly targets at MSCs that majorly form bone tissues in adult bone marrow [30] , [31] . Lepr-Cre;Mettl3 fl/fl mice recapitulated osteogenic block and adipogenic promotion seen in Prx1-Cre;Mettl3 fl/fl mice. Deletion of Mettl3 in Lepr + MSCs led to less trabecular bone in distal femoral, with a decrease in the number and thickness of trabeculae, as presented by lower BMD, BV/TV, Tb.N, and Tb.Th (Fig. 3a, b ). Histological examination revealed an increased abundance of adipose tissue in bone marrow milieu of Lepr-Cre;Mettl3 fl/fl mice in contrast to their Mettl3 fl/fl littermates (Fig. 3c, d ). Quantitative analysis of fat cells showed that both the fat cell number and density of the mutants increased more than doubled that of the controls (Fig. 3e ). Fig. 3 Deletion of Mettl3 in Lepr + MSCs results in bone impairment and marrow fat accumulation. a Representative μCT images of distal femurs of 4-month-old male mice. Scale bar, 500 μm. b Quantitative μCT analyses of distal end of femurs ( n = 8). c H&E staining of femoral sections from Mettl3 fl/fl and Lepr-Cre;Mettl3 fl/fl male mice. Scale bar, 500 μm. d Representative H&E staining of femur sections exhibiting the marrow adipose tissue. Scale bar, 50 μm. e Number and area of adipocytes in the distal marrow per tissue area ( n = 8). Data are expressed as mean ± s.e.m. ; * P < 0.05, ** P < 0.01, *** P < 0.001 by two-tailed Student’s t test Full size image Overexpression of Mettl3 prevents estrogen deficiency-induced osteoporosis Considering the pathologic effect of Mettl3 deletion in triggering osteoporosis, we questioned whether Mettl3 overexpression is capable to enhance skeletal health or prevent bone disorders. To this end, we generated the Prx1-Cre driven Mettl3-tdTomato knock-in mice ( Prx1-Cre;Mettl3 KI/KI ) to conditionally overexpress Mettl3 in MSCs (Supplementary Fig. 4a, b ). Prx1-Cre;Mettl3 KI/KI mice were viable and born at an expected Mendelian ratio. To study the potential protective role of Mettl3 overexpression in osteoporosis, 9-week-old Prx1-Cre;Mettl3 KI/KI female mice and their control littermates were subjected to ovariectomy (OVX), a classic model to induce the postmenopausal osteoporosis [32] , in which the estrogen deprivation upon postmenopause gave rise to imbalanced bone remodeling and increased marrow fat deposition [33] . Although Prx1-Cre;Mettl3 KI/KI mice did not exhibit significant change of bone mass in normal state, we observed a less decrease of trabecular bone density and bone volume in Mettl3 knock-in mice after OVX, compared to their controls (Fig. 4a, b ). The decline in Tb.N and Tb.Th, as well as the increase in Tb.Sp were less obvious when Mettl3 was overexpressed (Fig. 4b ). In addition, Mettl3 overexpression elevated osteoblast numbers in mice following OVX without affecting the osteoclast activity (Fig. 4 c-e). H&E staining and histomorphology analysis revealed an excessive accumulation of marrow adipocytes in ovariectomized control mice whilst the increase was minor in the ovariectomized Prx1-Cre;Mettl3 KI/KI mice (Fig. 4f, g ). Fig. 4 Overexpression of Mettl3 in MSCs prevents estrogen deficiency-induced osteoporosis. a Representative images of μCT reconstruction of distal femurs. Scale bar, 500 μm. b Quantitative μCT analyses of metaphysis region of distal femurs ( n = 8). c H&E staining of femoral sections from Mettl3 +l+ and Prx1-Cre;Mettl3 KI/KI female mice following sham and OVX. Scale bar, 500 μm. d TRAP staining of femur sections. Scale bar, 50 μm. e Histomorphometric analyses of distal femurs following sham and OVX ( n = 8). f Representative H&E staining of femur sections exhibiting the marrow adipose tissue. Scale bar, 50 μm. g Number and area of adipocytes in the distal marrow per tissue area ( n = 8). Data are expressed as mean ± s.e.m. ; * P < 0.05, ** P < 0.01, *** P < 0.001 by two-way ANOVA with Bonferroni post tests Full size image m 6 A regulates the translation of parathyroid hormone receptor-1 To dissect the underlying mechanism of Mettl3 in regulation of MSCs fate and bone formation, we performed the m 6 A MeRIP-Seq to identify the critical m 6 A targets in MSCs (Supplementary Data 1 ). As shown in Supplementary Figure 5a-c , the “GGAC” sequence motif is enriched in the m 6 A sites identified in MSCs (Supplementary Fig. 5a ), majority of the m 6 A sites are located in the CDS and the 3′UTR regions, with a small subset of peaks located in the 5′UTR and intron regions (Supplementary Fig. 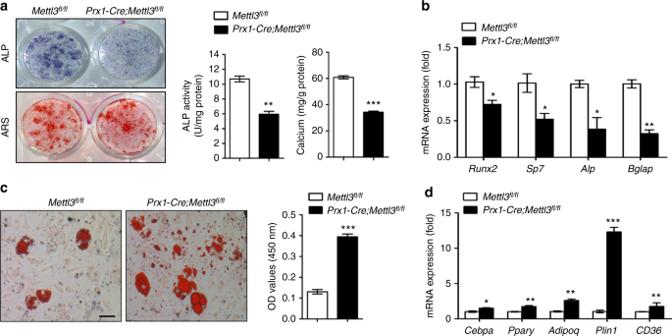Fig. 2 Mettl3-deficient MSCs exhibit compromised osteogenic potential and increased adipogenic differentiation.aRepresentative images and quantitative analyses of ALP and ARS staining of MSCs isolated fromMettl3fl/flandPrx1-Cre;Mettl3fl/flmice.bqRT-PCR analyses of the expression ofRunx2,Sp7,AlpandBglapunder osteogenic condition.cRepresentative images and quantitative analysis of oil red O staining. Scale bar, 100 μm.dqRT-PCR analyses of the expression ofCebpα,Pparγ,Adipoq, Plin1, andCD36under adipogenic condition. Results are from three independent experiments. Data are expressed as mean ± s.e.m.; *P< 0.05, **P< 0.01, ***P< 0.001 by two-tailed Student’sttest 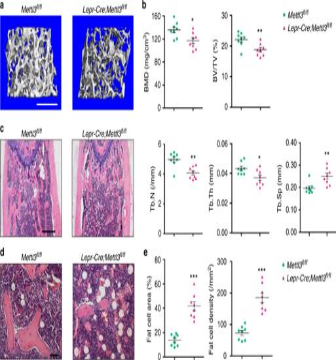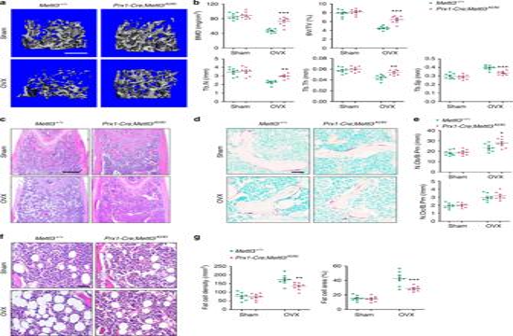Fig. 4 Overexpression ofMettl3in MSCs prevents estrogen deficiency-induced osteoporosis.aRepresentative images of μCT reconstruction of distal femurs. Scale bar, 500 μm.bQuantitative μCT analyses of metaphysis region of distal femurs (n= 8).cH&E staining of femoral sections fromMettl3+l+andPrx1-Cre;Mettl3KI/KIfemale mice following sham and OVX. Scale bar, 500 μm.dTRAP staining of femur sections. Scale bar, 50 μm.eHistomorphometric analyses of distal femurs following sham and OVX (n= 8).fRepresentative H&E staining of femur sections exhibiting the marrow adipose tissue. Scale bar, 50 μm.gNumber and area of adipocytes in the distal marrow per tissue area (n= 8). Data are expressed as mean ± s.e.m.; *P< 0.05, **P< 0.01, ***P< 0.001 by two-way ANOVA with Bonferroni post tests 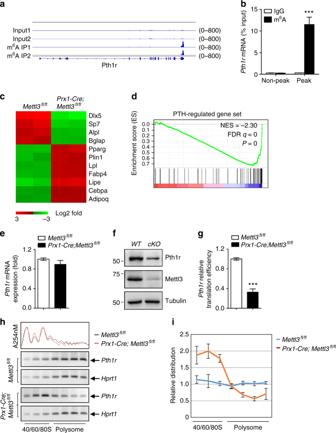Fig. 5 Mettl3-mediated m6A modification in MSCs regulates Pth1r translation.am6A MeRIP-Seq revealed thatPth1rhas high enriched and specific m6A peak near its translation stop codon.bMeRIP-qPCR validation ofPth1rm6A peak specificity.cHeatmap of representative osteogenesis and adipogenesis associated genes.dGSEA showed decreased enrichment of PTH-regulated genes inMettl3-deficient MSCs.eqRT-PCR analysis ofPth1rexpression.fWestern blot analysis of Pth1r.WT:Mettl3fl/fl,cKO:Prx1-Cre;Mettl3fl/fl.gTranslation efficiency of Pth1r.hPCR analysis ofPth1rmRNA in different polysome gradient fractions in theMettl3knockout and control cells. Hprt1 was used as a control.iQuantification ofPth1rmRNA relative distribution in theMettl3depleted and control cells. The band intensities ingwere analyzed by Image J. The relative amount ofPth1rorHprt1mRNA in each fraction was calculated as percentage of the total. Then the relative distribution ofPth1rmRNA was plotted by normalizing the percentage ofPth1rmRNA toHprt1mRNA in each fraction. Results are from three independent experiments. Data are expressed as mean ± s.e.m.; *P< 0.05, **P< 0.01, ***P< 0.001 by two-tailed Student’sttest Fig. 3 Deletion ofMettl3inLepr+MSCs results in bone impairment and marrow fat accumulation.aRepresentative μCT images of distal femurs of 4-month-old male mice. Scale bar, 500 μm.bQuantitative μCT analyses of distal end of femurs (n= 8).cH&E staining of femoral sections fromMettl3fl/flandLepr-Cre;Mettl3fl/flmale mice. Scale bar, 500 μm.dRepresentative H&E staining of femur sections exhibiting the marrow adipose tissue. Scale bar, 50 μm.eNumber and area of adipocytes in the distal marrow per tissue area (n= 8). Data are expressed as mean ± s.e.m.; *P< 0.05, **P< 0.01, ***P< 0.001 by two-tailed Student’sttest 5b ). Metagene analysis revealed that the m 6 A sites were predominantly localized near the translation stop codons (Supplementary Fig. 5c ). Furthermore, we found that Pth1r , a critical regulator of lineage allocation in MSCs and osteoblast precursors [34] , [35] , [36] , has high enriched and specific m 6 A peak near its translation stop codon (Fig. 5a, b ). Fig. 5 Mettl3-mediated m 6 A modification in MSCs regulates Pth1r translation. a m 6 A MeRIP-Seq revealed that Pth1r has high enriched and specific m 6 A peak near its translation stop codon. b MeRIP-qPCR validation of Pth1r m 6 A peak specificity. c Heatmap of representative osteogenesis and adipogenesis associated genes. d GSEA showed decreased enrichment of PTH-regulated genes in Mettl3 -deficient MSCs. e qRT-PCR analysis of Pth1r expression. f Western blot analysis of Pth1r. WT : Mettl3 fl/fl , cKO : Prx1-Cre;Mettl3 fl/fl . g Translation efficiency of Pth1r. h PCR analysis of Pth1r mRNA in different polysome gradient fractions in the Mettl3 knockout and control cells. Hprt1 was used as a control. i Quantification of Pth1r mRNA relative distribution in the Mettl3 depleted and control cells. The band intensities in g were analyzed by Image J. The relative amount of Pth1r or Hprt1 mRNA in each fraction was calculated as percentage of the total. Then the relative distribution of Pth1r mRNA was plotted by normalizing the percentage of Pth1r mRNA to Hprt1 mRNA in each fraction. Results are from three independent experiments. Data are expressed as mean ± s.e.m. ; * P < 0.05, ** P < 0.01, *** P < 0.001 by two-tailed Student’s t test Full size image Next, we carried out RNA sequencing (RNA-seq) to examine transcriptome profiles in MSCs isolated from Prx1-Cre;Mettl3 fl/fl mice and Mettl3 fl/fl controls, and confirmed the down-regulated expression of osteogenic marker genes, such as Dlx5 , Sp7 , Alpl , and Bglap , whereas upregulated expression of markers favoring adipocytic differentiation, including Pparg , Plin1 , and Fabp4 (Fig. 5c ). PTH1R is a key receptor of PTH and a parathyroid hormone-related protein (PTHrP) analog, abaloparatide, both are FDA-approved anabolic drugs for the treatment of osteoporosis [37] , [38] , and is indispensable for PTH’s function in modulating bone homeostasis [39] , [40] . To confirm that m 6 A modulates Pth1r, we preceded our RNA-seq data to gene set enrichment analysis (GSEA) using a published list of PTH-regulated genes [41] . We found that Mettl3 -deficient MSCs underwent a global down-regulation of PTH-regulated gene expression (Fig. 5d ), implying PTH/Pth1r signaling axis as a potential mechanism for Mettl3-mediated m 6 A methylation on MSCs fate. Both RNA-seq and quantitative RT-PCR showed that the mRNA expression of Pth1r was hardly affected by Mettl3 deletion (Fig. 5e ), whereas the Pth1r protein synthesis was inhibited upon Mettl3 deficiency as evidenced by western blot and decreased translation efficiency (Fig. 5f, g ), suggesting that m 6 A methylation affected Pth1r expression at translation level. We subsequently performed sucrose gradient centrifugation to resolve polysome fractions of Mettl3 knockout and control MSCs, and used RT-PCR to examine the distribution of endogenous Pth1r mRNA in different ribosome fractions. Our data revealed that the relative distribution of Pth1r mRNA was shifted from the polysome fractions to the sub-polysome fractions in Mettl3 knockout cells, indicating that Mettl3 depletion results in the decreased translation efficiency of Pth1r mRNA (Fig. 5h, i ). m 6 A is essential for PTH function Since Pth1r protein synthesis was hampered by Mettl3 depletion, we next examined physiological functions of PTH/Pth1r axis upon Mettl3 deficiency. Cyclic AMP-dependent protein kinase A (PKA) and extracellular signal-regulated kinases (ERK) pathways are important downstream pathways that mediate the intracellular signals and physiological responses during the anabolic effect of PTH [42] , [43] . Loss of Mettl3 attenuated the PTH-induced cAMP accumulation of Prx1-Cre;Mettl3 fl/fl MSCs (Fig. 6a ) and consequently inhibited the downstream phosphorylation of cAMP response element-binding protein (CREB) (Fig. 6b ). Meanwhile, despite having the same basal level of ERK1/2 as the control MSCs, mutant MSCs failed to activate the ERK1/2 pathway after PTH treatment (Fig. 6b ). Fig. 6 Deletion of Mettl3 exhibits inert responses to PTH treatment. a PTH-induced accumulation of cAMP in MSCs. Results are from three independent experiments. b Western blot analysis of p-ERK1/2, ERK1/2, p-CREB, and CREB. WT : Mettl3 fl/fl , cKO : Prx1-Cre;Mettl3 fl/fl . c Representative μCT images of distal femurs following PTH treatment. d Quantitative μCT analyses of metaphysis region of distal femurs ( n = 8). e H&E staining of femoral sections from Mettl3 fl/fl and Prx1-Cre;Mettl3 fl/+ female mice following PTH treatment. Scale bar, 500 μm. f TRAP staining of femur sections. Scale bar, 50 μm. g Histomorphometric analyses of distal femurs following PTH treatment ( n = 8). h Representative H&E staining of femur sections exhibiting the marrow adipose tissue. Scale bar, 50 μm. i Number and area of adipocytes in the distal marrow per tissue area ( n = 8). Data are expressed as mean ± s.e.m. ; * P < 0.05, ** P < 0.01, *** P < 0.001 by two-way ANOVA with Bonferroni post tests Full size image To investigate the potential role of Mettl3 in PTH-mediated bone remodeling in vivo, we performed intermittent PTH (1-34) injection to 3-month-old Mettl3 fl/fl and Prx1-Cre;Mettl3 fl/+ female mice to compare their responses to PTH treatment. In contrast with the sharp growth of trabecular bone mass in Mettl3 fl/fl controls, there were only slight changes in the BMD, BV/TV, Tb.N and Tb.Sp in the Prx1-Cre;Mettl3 fl/+ mice (Fig. 6c, d ). Furthermore, Prx1-Cre;Mettl3 fl/+ mice failed to undergo an effective increase in bone remodeling after PTH treatment (Fig. 6e–g ), confirming that Mettl3 knockout blunted PTH-induced osteogenic effects. Besides a marked enrichment in osteogenesis, PTH also inhibits adipocytic differentiation to promote bone formation [35] , [44] . In our experiment, PTH injection significantly reduced MAT accumulation in Mettl3 fl/fl mice whilst hardly reversing the high marrow adiposity in Prx1-Cre;Mettl3 fl/+ mice (Fig. 6h, i ), consolidating our findings that m 6 A affects both osteogenic and adipogenic differentiation of MSCs by regulating PTH/Pth1r signaling axis. Overexpression of Pth1r partially rescues the proper lineage commitment of Mettl3 -deficient MSCs Next, we transduced adenoviral constructs overexpressing Pth1r (Ad- Pth1r ), or gfp (Ad- gfp ) as a control, into Prx1-Cre;Mettl3 fl/fl MSCs. Ad- Pth1r successfully restored the protein level of Pth1r in Prx1-Cre;Mettl3 fl/fl MSCs (Fig. 7a ), and significantly improved the ALP activity and calcium nodule formation (Fig. 7b, c ). Furthermore, Pth1r overexpression ameliorated the increased intensity of oil red O staining arising from m 6 A reduction (Fig. 7e ). qRT-PCR analysis also revealed an up-regulation of osteogenic markers along with a down-regulation of adipogenic markers after Pth1r transduction (Fig. 7d, f ). These data demonstrate that Pth1r overexpression is able to partially rescue the proper lineage commitment of Mettl3 -deficient MSCs. Fig. 7 Overexpression of Pth1r ameliorates osteogenic differentiation of Mettl3 -deficient MSCs. a Western blot analysis of Pth1r and Mettl3. WT : Mettl3 fl/fl , cKO : Prx1-Cre;Mettl3 fl/fl . b , c Representative images and quantitative analyses of ALP and ARS staining. d qRT-PCR analyses of the expression of Runx2 , Sp7 , Alp , and Bglap under osteogenic condition. e Representative images and quantitative analysis of oil red O staining. Scale bar, 100 μm. f qRT-PCR analyses of the expression of Cebpα , Pparγ , Adipoq, Plin1 and CD36 under adipogenic condition. Results are from three independent experiments. Data are expressed as mean ± s.e.m. ; * P < 0.05, ** P < 0.01, *** P < 0.001 ( c , e ) and a: P < 0.05, b: P < 0.01, c: P < 0.001 ( d , f ) by one-way ANOVA with Tukey’s post hoc test Full size image Mettl3-mediated m 6 A modification in eukaryotic RNA has a broad functional influence on stabilizing homeostasis, while any perturbation in m 6 A levels can result in malfunction or diseases. Recent studies have consecutively revealed a strong and intricate relation of m 6 A modification with stem cell regulation. Mis-regulated m 6 A level disrupted the timely controlled embryonic stem cell differentiation [20] , [21] , impaired the normal generation and differentiation of hematopoietic stem cells [23] , [24] as well as inhibiting functional development of neurogenesis, spermatogenesis, and T cell homeostasis [25] , [26] , [27] , [28] , [45] . Using different temporal MSCs markers, Prx1 and Lepr , we generated two genetic murine models to conditionally knockout Mettl3 from early limb bud mesenchyme and adult bone marrow, respectively. We showed that deletion of Mettl3 in bone marrow MSCs disrupts cell fate in mice and results in osteoporosis pathological phenotypes such as decreased bone mass with incompetent osteogenic potential, and increased marrow adiposity with enhanced adipogenic potential, uncovering an efficient and specific regulation of m 6 A on MSCs. Furthermore, Mettl3 gain-of-function prevents estrogen deficiency-induced postmenopausal osteoporosis, establishing the indispensability of Mettl3 in defining bone marrow MSC’s fate and thereby ensuring skeletal health. Accumulating evidences have pointed out the regulatory role of m 6 A in translation. In cooperation with m 6 A readers, m 6 A facilitates translation initiation, and responds to selective mRNA translation under heat shock stress [14] , [16] , [46] , [47] , [48] . Alterations in translation efficiency of m 6 A marked transcripts affected normal hematopoiesis [23] , [24] and mammalian spermatogenesis [28] , [49] . Here we discover that m 6 A is essential for Pth1r translation. Loss of Mettl3 caused strong shift of Pth1r mRNA from the polysome fractions to the sub-polysome fractions, therefore slowing down the protein synthesis of Pth1r and further blocking the downstream signaling pathways of Pth1r responsive to PTH treatment. Intermittent PTH treatment promotes bone formation, which is achieved by increasing osteoblasts number, delaying osteoblast apoptosis, activating bone-lining cells and reducing marrow fat [34] , [42] , [44] . PTH1R is a direct signaling mediator of PTH in promoting osteoblastic lineage of MSCs while aberrant PTH1R expression can lead to MAT accumulation as a consequence of preferential adipogenic differentiation [34] , [35] , [50] . Mettl3 knockout reduced the global methylation level of m 6 A in mice and significantly impaired Pth1r function. The persistence in high marrow adiposity and the poorly elevated bone mass in m 6 A deficient mice following intermittent PTH(1-34) injection supported a blunt response to PTH anabolic effect. Our subsequent finding that overexpression of Pth1r could largely reverse skewed MSCs differentiation towards adipocytes and improve osteogenesis further confirmed PTH/Pth1r signaling pathway as a novel mechanism whereby Mettl3-mediated m 6 A modification controls the lineage allocation of MSCs. PTH also stimulates osteoclast formation and activity by increasing the receptor activator of nuclear factor κ-B ligand (RANKL)/osteoprotegerin (OPG) ratio through its receptor [51] , [52] , [53] . Although the protein synthesis of Pth1r was largely compromised upon Mettl3 ablation in our study, we found that the number of osteoclasts was rather elevated. One explanation for this increase in osteoclasts, we presume, is that Mettl3 has another relevant target in bone cells besides Pth1r, since our overexpression of Pth1r has only achieved a partial rescue. Another possible explanation is that the adipogenic favored differentiation of MSCs upon Pth1r malfunction promotes osteoclast activity. 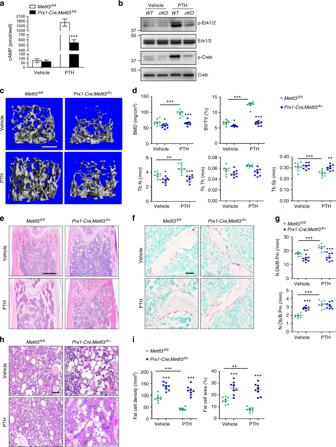Fig. 6 Deletion ofMettl3exhibits inert responses to PTH treatment.aPTH-induced accumulation of cAMP in MSCs. Results are from three independent experiments.bWestern blot analysis of p-ERK1/2, ERK1/2, p-CREB, and CREB.WT:Mettl3fl/fl,cKO:Prx1-Cre;Mettl3fl/fl.cRepresentative μCT images of distal femurs following PTH treatment.dQuantitative μCT analyses of metaphysis region of distal femurs (n= 8).eH&E staining of femoral sections fromMettl3fl/flandPrx1-Cre;Mettl3fl/+female mice following PTH treatment. Scale bar, 500 μm.fTRAP staining of femur sections. Scale bar, 50 μm.gHistomorphometric analyses of distal femurs following PTH treatment (n= 8).hRepresentative H&E staining of femur sections exhibiting the marrow adipose tissue. Scale bar, 50 μm.iNumber and area of adipocytes in the distal marrow per tissue area (n= 8). Data are expressed as mean ± s.e.m.; *P< 0.05, **P< 0.01, ***P< 0.001 by two-way ANOVA with Bonferroni post tests 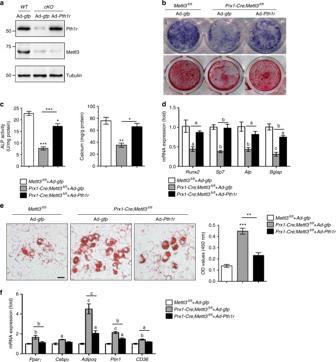Fig. 7 Overexpression ofPth1rameliorates osteogenic differentiation ofMettl3-deficient MSCs.aWestern blot analysis of Pth1r and Mettl3.WT:Mettl3fl/fl,cKO:Prx1-Cre;Mettl3fl/fl.b,cRepresentative images and quantitative analyses of ALP and ARS staining.dqRT-PCR analyses of the expression ofRunx2,Sp7,Alp, andBglapunder osteogenic condition.eRepresentative images and quantitative analysis of oil red O staining. Scale bar, 100 μm.fqRT-PCR analyses of the expression ofCebpα,Pparγ,Adipoq, Plin1andCD36under adipogenic condition. Results are from three independent experiments. Data are expressed as mean ± s.e.m.; *P< 0.05, **P< 0.01, ***P< 0.001 (c,e) and a:P< 0.05, b:P< 0.01, c:P< 0.001 (d,f) by one-way ANOVA with Tukey’s post hoc test Fan et al. demonstrated in their recent study that bone marrow adipocytes are the source of RANKL in the absence of PTH1R signaling [34] . Similar to their finding, our TRAP staining showed that osteoclasts in Mettl3 mutant mice were located very near to the large adipocytes (Fig. 1d ). Therefore, we speculated that the excessive accumulated marrow adipose tissue in Mettl3 conditional knockout mice may also account for the increase of osteoclast number. Of note, unlike the severe chondrodysplasia in Prx1-Cre;PTH1R fl/fl mice reported by Fan et al. [54] , we observed only slight yet not significant growth plate cellular architecture changes in Prx1-Cre;Mettl3 fl/fl mice. Our finding that Mettl3 does not express in growth plate chondrocytes, thus may not participate in chondrogenesis, can be an explanation for this discrepancy in growth plate phenotype. The minute difference in hypertrophic zone between Prx1-Cre;Mettl3 fl/fl mice and their controls might due to an indirect effect of Pth1r impairment in Mettl3 -depleted osteoblasts, which further affects endochondral vascularization in the growth plate [55] . In summary, we demonstrate that reduced epigenetic modification of m 6 A in bone marrow MSCs from an early phase inhibits Pth1r translation in mammals and blocks their anabolic responses to PTH during bone accrual. These functional defects tilt the delicate MSC differentiation balance toward adipogenic lineage, causing severe bone loss and excessive MAT accumulation. Our data enrich the evidence of m 6 A in modulating stem cell differentiation, and uncover the functional link between mis-regulated m 6 A modification and bone pathological disorders, therefore may shed light on the development of new therapeutic strategies for osteoporosis. Generation of conditional Mettl3 knockout and knock-in mice For conditional knockout, Mettl3 f l/+ mice with C57BL6/J background were generated using CRISPR-Cas9 systems [56] , [57] . Briefly, the exon 2 and exon 3 of Mettl3 is the target of interest in generation of conditional knockout floxed Mettl3 allele. With the help of a CRISPR design tool ( http://crispr.mit.edu ), sgRNAs were designed to recognize a region either upstream or downstream of the target, and then were screened for on-target activity using a Universal CRISPR Activity Assay (UCA TM , Biocytogen Inc, Beijing). Donor vectors structured with the Lox P flanked exon 2 and exon 3 was mixed with Cas9 mRNA and sgRNAs and co-injected into the cytoplasm of one-cell stage fertilized C57BL6/J eggs. The injected zygotes were then transferred into oviducts of Kunming pesudopregnant females to obtain F0 mice. Tail genomic DNA PCR and sequencing were performed to identify F0 mice with expected genotype, which were afterwards crossed with C57BL6/J mice to establish germline-transmitted F1 founders. Both PCR genotyping and southern blot were applied to ensure the correct genotype of generated Mettl3 fl/+ mice. For conditional knock-in, CRISPR-Cas9 techniques were also performed. The targeting vector consisting of a loxP flanked stop codon regulatory element and a downstream Mettl3 coding sequence (CDS) was inserted into wild type Rosa26 allele to obtain the targeted conditional Mettl3 knock-in allele. We designed a tdTomato sequence at the downstream of Mettl3 CDS to facilitate our verification of knock-in efficiency later in the research. The targeted allele was then reconstructed into a plasmid under the mediation of Cas9/sgRNAs. After the co-injection of the reconstructed plasmid into fertilized C57BL6/J eggs, PCR genotyping and southern blot were executed to obtain desirable F1 mice that were recombined with targeted Mettl3 knock-in alleles. Prx1-Cre and Lepr-Cre transgenic mice were purchased from The Jackson Laboratory. We crossed male Prx1-Cre or Lepr-Cre mice with Mettl3 f l/+ mice to obtain Prx1-Cre;Mettl3 fl/+ mice and Lepr-Cre;Mettl3 fl/+ mice as heterozygous conditional Mettl3 knockout. By mating Prx1-Cre;Mettl3 fl/+ or Lepr-Cre;Mettl3 fl/+ male mice with Mettl3 f l/+ female mice, we obtained Prx1-Cre;Mettl3 fl/fl mice and Lepr-Cre;Mettl3 fl/fl mice as homozygous conditional Mettl3 knockout mice. The same mating strategy was used in the generation of conditional Mettl3 knock-in mice. The genotype of transgenic mice was identified by PCR analyses of genomic DNA extracted from mouse tails. Primers for floxed Mettl3 knockout allele genotyping were forward (5′-TCCCTGGGAAACATAATCACATCC-3′) and reverse (5′-CTTCTCCTCCTCTCAAATGATACAAT-3′). Primers for floxed Mettl3 knock-in allele genotyping were forward (5′-AGTCGCTCTGAGTTGTTATCAG-3′), wild-type band reverse (5′-TGAGCATGTCTTTAATCTACCTCGATG-3′), mutant band reverse (5′- AGTCCCTATTGGCGTTACTATGG-3′). Primers for Cre transgene genotyping were wild-type band forward (5′-CCATCTGCCACCAGCCAG-3′), wild-type band reverse (5′-TCGCCATCTTCCAGCAGG-3′), mutant band forward (5′-ACTGGGATCTTCGAACTCTTTGGAC-3′), and mutant band reverse (5′-GATGTTGGGGCACTGCTCATTCACC-3′). All the mice were bred and maintained under specific-pathogen-free conditions. All studies performed were approved by the Subcommittee on Research and Animal Care (SRAC) of Sichuan University. LC-MS/MS analysis of m 6 A level The integrity and quantity of each total RNA samples extracted from primary MSCs was examined using agarose gel electrophoresis and Nanodrop™ instrument. mRNA was isolated from total RNA using NEBNext® Poly(A) mRNA Magnetic Isolation Module (For next generation sequencing using). Purified mRNA was quantified using NanoDrop ND-1000. mRNA was hydrolyzed to single nucleosides and then nucleosides were dephosphorylated by enzyme mix. Pretreated nucleosides solution was deproteinized using Satorius 10,000-Da MWCO spin filter. Analysis of nucleoside mixtures was performed on Agilent 6460 QQQ mass spectrometer with an Agilent 1290 HPLC system. Multi reaction monitoring (MRM) mode was performed because of its high selectivity and sensitivity attained working with parent-to-product ion transitions. LC-MS/MS data was acquired using Agilent Qualitative Analysis software. MRM peaks of each modified nucleoside were extracted and normalized to peak areas of normal adenosine in each samples. Samples were run in duplicate, and m 6 A/A ratios were calculated. μCT and histomorphometric analyses The harvested bone tissues were fixed in 4% polyoxymethylene for 2 days and then stored in 70% ethanol at 4 °C before being processed. μCT analysis was performed according to recent guidelines [58] using a μCT 80 microCT system (Scanco Medical, Bassersdorf, Switzerland) with a spatial resolution of 8 μm (55 kV, 114 mA, 500 ms integration time). For the analysis of cortical bone regeneration, the volume of interest (VOI) was defined as a cylindrical area covering the initial bone defect. Bone volume (BV/TV) was calculated within the delimited VOI. Processing of undecalcified bone specimens and cancellous bone histomorphometry were performed as described [59] , [60] . Followed by microCT scanning, femurs were dehydrated and embedded in methylmethacrylate. Five‐µm‐thick sections were prepared using a Leica RM2235 microtome and were stained by the von Kossa/nuclear fast red method. Histomorphometric measurements in the distal end of femurs were made using OsteoMeasure software (OsteoMetrics, Decatur, GA). Immunohistochemical staining The dissected femurs were fixed in 4% polyoxymethylene for 2 days and decalcified in 10% EDTA for 2 weeks before sectioning (5 μm). Slides were subjected to sodium citrate buffer at 99 °C for 20 min for antigen retrieval and then incubated with rabbit anti-METTL3/MT-A70 (1:200, Bethyl, Cat No: A301-567A), or rabbit polyclonal anti-FABP4 (1:200, Abcam, Cat No: ab13979). Ovariectomy Nine-week-old female conditional Mettl3 knock-in mice and littermate controls were selected for ovariectomy and randomly assigned to OVX or sham group. Ovaries were surgically removed on both sides after anesthesia [61] . In short, small dorsal incisions below the bottom of the rib cage were made to penetrate the skin and muscles respectively. After locating the ovary, we exposed the oviduct and ligated it before the removal of the ovary. For sham group, ovaries were replaced back into the peritoneal cavity directly after their locating. Finally, we sutured the wound and bred the operated mice in sham and OVX group for another 5 weeks before sacrifice. Cell culture We isolated primary MSCs by flushing the bone marrow of tibiae and femurs. The cells were then cultured in α-MEM (Hyclone) supplemented with 10% fetal bovine serum (Gibco),100 units/ml penicillin (Gibco) and 100 μg/ml streptomycin (Gibco), at 37 °C with an atmosphere of 5% CO 2 and 95% humidity. For osteogenic induction, MSCs were seeded in six-well plates and treated with osteogenic medium containing 50 μg/ml ascorbic acid, 5 mM β-glycerophosphate, and 100 nM dexamethasone (all from Sigma). For adipogenic induction, MSCs were seeded in six-well plates and treated with adipogenic medium containing 0.5 μM isobutylmethylxanthin (Sigma), 10 μg/ml insulin (Sigma), and 1 μM dexamethasone (Sigma). ALP, alizarin red staining, and oil red O staining For ALP staining, cells were fixed after 10 days induction of osteogenic differentiation with 4% polyoxymethylene for 15 min and incubated with 0.1 M Tris buffer (pH 9.3) containing 0.25% naphthol AS-BI phosphate (Sigma) and 0.75% Fast Blue BB (Sigma). Quantitative ALP activity was performed with a commercial kit according to the manufacturer’s protocol (Cell Biolab, San Diego, CA). The optical density was determined by a spectrophotometer (Thermo Fisher Scientific) at 450 nm. For alizarin red staining (ARS) staining, cells were fixed after 10 days induction of osteogenic differentiation with 4% polyoxymethylene for 15 min and stained with 1% Alizarin red S (pH 4.2, Sigma-Aldrich) for 5 min. Mineralized matrix stained with alizarin red were destained with 10% cetylpyridinium chloride in 10 mM sodium phosphate (pH 7.0), and the calcium concentration was determined by a spectrophotometer (Thermo Fisher Scientific) at 562 nm using a standard calcium curve in the same solution [62] , [63] . For oil red O staining, after 2–3 weeks of adipogenic induction, cells were subjected to oil red O staining (Sigma) according to the manufacturer’s protocols. 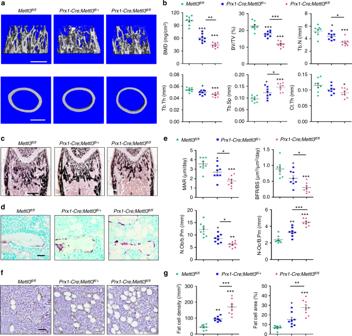The staining was then dissolved with isopropanol and quantified by a spectrophotometer (Thermo Fisher Scientific) at 450 nm, as described previously [34] . Quantitative RT-PCR Total RNA of cultured cells was extracted using Trizol (Invitrogen) according to manufacturer’s instruction. cDNA was prepared using PrimeScript RT reagent Kit with gDNA Eraser (Takara). The RNA concentration was measured with a NanoDrop 2000 (Thermo Fisher Scientific). qRT-PCR was performed using SYBR Premix Ex Taq II (Takara) in CFX96 Real-Time System (Bio-Rad). Relative gene expression was normalized by Gapdh for osteogenic differentiation and 36B4 for adipogenic differentiation using a 2 −ΔΔCt method. Fig. 1 Deletion ofMettl3in MSCs leads to low bone mass and high marrow adiposity.aRepresentative μCT images of distal femurs and midshaft cortical bone. Scale bar, 500 μm.bQuantitative μCT analyses of distal end of femurs (n= 8).cVon Kossa staining of undecalcified sections of femurs. Scale bar, 500 μm.dTRAP staining of femur sections. Scale bar, 50 μm.eHistomorphometric analyses of trabecular bone from the femur metaphysic (n= 8).fImmunohistochemical staining of FABP4. Scale bar, 50 μm.gNumber and area of adipocytes in the distal marrow per tissue area (n= 8). Data are expressed as mean ± s.e.m.; *P< 0.05, **P< 0.01, ***P< 0.001 by one-way ANOVA with Tukey’s post hoc test The primers are listed in Supplementary Table 1 . Western blot Cells were lysed in RIPA buffer (Pierce, Rockford, IL) on ice. For PTH treatment group, cells were given 100 nM human recombinant PTH (1-34) (Bachem, Torrance, CA, USA) at 37 °C for 30 min prior to sampling. The samples were heated at 95 ℃ for 5 min in sample buffer containing 2% SDS and 1% 2-mercaptoethanol, separated on 10% SDS–polyacrylamide gels, and transferred to PVDF membranes by a wet transfer apparatus (Bio-Rad). The membranes were blotted with 5% BSA for 1 h and then incubated overnight with rabbit METTL3 polyclonal antibody (1:1000, Proteintech, Cat No: 15073-1-AP), PTH1R antibody (1:1000, Assay Biotechnology, Cat No: G220), p44/42 MAPK (Erk1/2) rabbit mAb (1:1000, Cell signaling, Cat No: 4695), phospho-p44/42 MAPK (Erk1/2) rabbit mAb (1:2000, Cell signaling, Cat No: 4370), CREB rabbit mAb (1:1000, Cell signaling, Cat No: 9197), phospho-CREB rabbit mAb (1:1000, Cell signaling, 9198), α-tubulin rabbit polyclonal antibody (1:2000, Beyotime, Cat No: AF0001), followed by incubation with a goat anti-rabbit IgG secondary antibody HRP conjugated (1:5000, Signaling antibody, Cat No: L3012-2). The antibody-antigen complexes were visualized with Immobilon reagents (Millipore). The uncropped gel images are shown in Supplementary Fig. 6 . m 6 A MeRIP-Seq (methylated RNA immunoprecipatation and sequencing) The MSC m 6 A MeRIP-Seq and data analysis were performed as previously described [64] , [65] . Briefly, Trizol reagent was used for the isolation of total RNA from MSC, and then the PolyATtract mRNA Isolation System IV (Promega Z5310) was used to enrich mRNA from MSC total RNA sample. Two μg of the purified mRNA was fragmentized into about 100 nt length with ZnCl 2 buffer at 94 °C for 5 min. The mRNA fragments were purified with Oligo Clean & Concentrator TM (Zymoresearch D4061) and then subjected to immunoprecipitation with α-m 6 A antibody (1:100, Synaptic Systems, Cat No: 202003). After extensive wash, the methylated fragments were eluted by competition using free N 6 -Methyladenosine (Santa Cruz Biotechnology, sc-215524) and then used for library construction with the TruSeq Stranded mRNA Sample Prep Kits (Illumina RS-122-2101). The input and m 6 A MeRIP libraries were sequenced with Illumina NextSeq 500 with high output kit. The sequence reads mapping, peak calling and visualization, metagene analysis of m 6 A distribution, motif search and gene ontology analysis were performed as previously described [65] . RNA-seq and gene set enrichment analysis Total RNAs from MSCs of Prx1-Cre;Mettl3 fl/fl mice and their control littermates were extracted by Trizol reagent and purified using poly-T oligo-attached magnetic beads. Sequencing libraries were generated using NEBNext® Ultra™ RNA Library Prep Kit for Illumina® (NEB, USA) following manufacturer’s recommendations, and were then subjected to Illumina HiSeq 2500. We used FastQC (v0.11.5) and FASTX toolkit (0.0.13) to control the quality of RNA-seq data and mapped them to Mus musculus reference genomes using HISAT2 (v.2.0.4). Ballgown software (v.3.4.0) was performed to identify differentially expressed genes and transcripts. Genes were considered significantly differentially expressed if showing ≥2.0 fold change and P value < 0.05. For GSEA, PTH-regulated gene list was obtained from a published study [41] . GSEA were performed with GSEA software ( http://www.broad.mit.edu/GSEA ) as previously described [66] . In short, we first imported our gene list of interest into the software and examined whether this given gene set showed statistically significant, concordant differences between two biological states (for example, phenotypes). P values were computed using a bootstrap distribution created by resampling gene sets of the same cardinality. Polysome fractionation and RT-PCR Cells were washed with ice old PBS twice and then PBS containing 100 μg/ml Cycloheximide was added to the cell culture dishes to stop translation. Cells were scraped and lyzed with cell extraction buffer to collect the cytoplasmic extracts, which were loaded onto the top of 11 ml 10–50% sucrose gradient tube. The sucrose gradient tubes were centrifuged at 222,000 × g with SW41Ti rotor for 2 h and 30 min at 4 °C. Then the ribosome fractions were collected using the ISCO gradient fractionators, with measurement of absorbance at 254 nm. RNA samples were isolated from different fractions using Trizol and reverse transcription and PCR were performed as previously described to determine the relative distribution of Pth1r mRNA in different ribosome fractions [65] . cAMP assay Cells were cultured in six-well plates and stimulated with vehicle or 100 nM human recombinant PTH (1-34) (Bachem, Torrance, CA, USA) at 37 °C for 15 min [67] . We then carried out the cAMP assay using the cAMP Biotrak Enzymeimmunoassay (EIA) System (GE Healthcare Bio-Science Corp., Piscataway, NJ, USA) and followed the manufacturer’ s instruction. Intermittent PTH (1-34) injection Subcutaneous daily injection of 80 μg/kg of human recombinant PTH (1-34) (Bachem, Torrance, CA, USA) was given to 12-week-old female Prx1-Cre;Mettl3 fl/+ and control mice for 4 weeks. An equal volume of sterile saline was given to animals in the vehicle group. The assignment of Prx1-Cre;Mettl3 fl/+ and control mice into PTH or vehicle group was randomized. Adenoviral infection Adenoviruses encoding mouse Pth1r gene and/or green fluorescent protein (GFP) were obtained from Cyagen. Primary MSCs isolated from bone marrow of tibiae and femurs were infected with Ad- Pth1r or Ad- gfp for 12 h at 37 °C with an atmosphere of 5% CO 2 and 95% humidity. Statistical analysis All data were expressed as mean ± s.e.m. Statistical differences were analyzed by unpaired two-tailed Student’s t test for comparison between two groups, one-way ANOVA followed by Tukey’s post hoc test for multiple comparisons, and two-way ANOVA followed by Bonferroni post test for comparison between sham and OVX groups, as well as vehicle and PTH treatment groups. A P value <0.05 was considered to be statistically significant.